Interplay between glucose and leptin signalling determines the strength of GABAergic synapses at POMC neurons Regulation of GABAergic inhibitory inputs and alterations in POMC neuron activity by nutrients and adiposity signals regulate energy and glucose homeostasis. Thus, understanding how POMC neurons integrate these two signal molecules at the synaptic level is important. Here we show that leptin’s action on GABA release to POMC neurons is influenced by glucose levels. Leptin stimulates the JAK2–PI3K pathway in both presynaptic GABAergic terminals and postsynaptic POMC neurons. Inhibition of AMPK activity in presynaptic terminals decreases GABA release at 10 mM glucose. However, postsynaptic TRPC channel opening by the PI3K–PLC signalling pathway in POMC neurons enhances spontaneous GABA release via activation of presynaptic MC3/4 and mGlu receptors at 2.5 mM glucose. High-fat feeding blunts AMPK-dependent presynaptic inhibition, whereas PLC-mediated GABAergic feedback inhibition remains responsive to leptin. Our data indicate that the interplay between glucose and leptin signalling in glutamatergic POMC neurons is critical for determining the strength of inhibitory tone towards POMC neurons. Leptin is an adipocyte-derived hormone whose actions are required for normal energy homeostasis [1] , [2] . Among leptin-responsive areas in the brain, leptin receptors (LepRs) are particularly highly expressed in the arcuate nucleus of the hypothalamus (ARC) [3] , [4] . The ARC contains proopiomelanocortin (POMC) neurons that are a critical regulator for energy balance and glucose homeostasis [5] , [6] . Mice with targeted deletion of the Pomc gene and their cognate receptors MC3/4R are obese [7] , [8] , [9] , [10] . Moreover, abnormalities in POMC synthesis and processing as well as defects in the action of POMC-derived peptides cause obesity in humans [11] , [12] , [13] , [14] . Hence, dysregulation in melanocortin signalling leads to obesity and metabolic disorders in animals and humans. There are extensive studies on the regulation of POMC neurons by nutrients and circulating adiposity signals including glucose and leptin. Leptin depolarizes POMC neurons via activation of canonical transient receptor potential (TRPC) channels [15] . Activation of TRPC channels is mediated by the janus kinase 2 (JAK2)–phosphatidylinositide 3-kinases (PI3K)–phospholipase C (PLC) pathway [15] . This JAK2–PI3K–PLC pathway in POMC neurons plays an essential role in the regulation of energy and glucose homeostasis. For instance, in mice with POMC-specific ablation of phosphatidylinositol 3,4,5-trisphosphate phosphatase (Pten), which promotes continuous activation of the PI3K pathway, leptin is not able to elicit action potentials, although leptin stimulates signal transducer and activator of transcription 3 (STAT3) phosphorylation [16] . Furthermore, disruption of PI3K in POMC neurons blunts leptin’s action on the membrane potential as well as food intake, although mice show normal long-term body weight regulation [17] . This is further supported by the study showing that mice deficient of the p110β isoform of PI3K in POMC neurons exhibit leptin resistance, increased adiposity and increased food intake, associated with no electrical response to leptin [18] . Although the JAK2–STAT3 pathway contributes to the regulation of long-term energy homeostasis via the transcription of POMC and the inhibitory suppressor of cytokine signalling 3 (refs 19 , 20 , 21 ), the JAK2–PI3K pathway appears to be important in the regulation of POMC neuron activity, resulting in leptin-induced hypophagia. Kahn and colleagues [22] demonstrated another important signalling pathway that is required for leptin’s anorexigenic effects. Leptin decreases the activity of the α2 subunit of adenosine monophosphate-activated protein kinase (AMPK) via phosphorylation of AMPK α subunits. This appears to be a key downstream target of the JAK2–PI3K pathway [22] , [23] . High-fat feeding suppresses basal AMPK activity in the hypothalamus and, more importantly, leptin fails to attenuate hypothalamic AMPK activity in diet-induced obese mice [24] . Interestingly, POMC neurons from the animals deficient for the α2 subunit of AMPK in POMC neurons remain responsive to leptin, but do not respond to alterations in extracellular glucose levels [25] . Hence, ARC neurons integrate nutrients and adiposity signals through alterations in AMPK activity. Alterations in POMC neuron activity by glucose and leptin modulate the release of α-melanocyte-stimulating hormone (α-MSH) [26] , [27] . Importantly, there exists an autoinhibitory loop from melanocortin peptides in POMC neurons [28] . We thus investigated whether leptin signalling in ARC POMC neurons is influenced by glucose levels. In this study, leptin’s inhibitory effect on spontaneous GABA (γ-aminobutyric acid) release at 10 mM glucose is completely absent at 2.5 mM glucose. Rather the effect of leptin on GABA release is stimulatory at 2.5 mM glucose. Reduced GABA release is owing solely to the inhibition of presynaptic AMPK activity. However, LepR activation on POMC neurons opens TRPC channels via the JAK2–PI3K–PLC pathway. Calcium entry through TRPC channels induces the release of α-MSH and glutamate. Activation of presynaptic MC3/4 and metabotropic glutamate (mGlu) receptors enhances GABA release. High-fat feeding elevates the JAK2–PI3K–PLC signalling pathway, while reducing AMPK activity in POMC neurons. Hence, GABAergic synapses at POMC neurons integrate glucose and leptin signalling, and this integration is subject to modulation by high-fat feeding. Two distinct effects of leptin on GABAergic sIPSCs This report is based on recordings from ~500 neurons in acute hypothalamus slices from both male and female animals. We examined whether alterations in extracellular glucose levels influence leptin’s action on spontaneous GABAergic inhibitory currents (sIPSCs) to POMC neurons. As described in the prior studies [28] , [29] , leptin (100 nM) significantly depressed GABAergic transmission in a subset of POMC neurons at 10 mM glucose, consistent with a prior study [28] ( Fig. 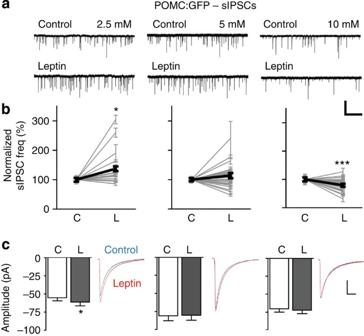Figure 1: Two distinct effects of leptin on sIPSCs. (a) Representative recording traces showing sIPSCs recorded from POMC neurons at different glucose levels. Addition of leptin (100 nM) robustly increased sIPSC frequency at 2.5 mM glucose, whereas leptin had an inhibitory effect on sIPSCs at 10 mM glucose. HP=−70 mV. Scale bar, 100 pA, 10 s. (b) Graphs showing normalized frequency of sIPSCs from individual POMC neurons before and after treatment with leptin (100 nM) at different glucose levels (bold line, total mean change in sIPSC frequency; 2.5 mM,n=19 neurons; 5 mM,n=27 neurons; 10 mM,n=26 neurons). C, control; L, leptin. (c) Pooled data showing sIPSC amplitude. Superimposition of traces of sIPSCs before (blue) and after (red) application of leptin. Leptin increased the mean amplitude of sIPSCs at 2.5 mM glucose (2.5 mM,n=19 neurons; 5 mM,n=27 neurons; 10 mM,n=26 neurons). Scale bar, 20 pA, 20 ms. *P<0.05, ***P<0.001 versus control (pairedt-test). All data are shown as mean±s.e.m. 1a,b and Table 1 ; the mean percent change in sIPSC frequency: 60.3±4.9% of control; n =11 out of 26 neurons). Treatment with leptin significantly reduced the mean frequency without altering the mean amplitude of sIPSCs ( Fig. 1c and Table 1 ). Figure 1: Two distinct effects of leptin on sIPSCs. ( a ) Representative recording traces showing sIPSCs recorded from POMC neurons at different glucose levels. Addition of leptin (100 nM) robustly increased sIPSC frequency at 2.5 mM glucose, whereas leptin had an inhibitory effect on sIPSCs at 10 mM glucose. HP=−70 mV. Scale bar, 100 pA, 10 s. ( b ) Graphs showing normalized frequency of sIPSCs from individual POMC neurons before and after treatment with leptin (100 nM) at different glucose levels (bold line, total mean change in sIPSC frequency; 2.5 mM, n =19 neurons; 5 mM, n =27 neurons; 10 mM, n =26 neurons). C, control; L, leptin. ( c ) Pooled data showing sIPSC amplitude. Superimposition of traces of sIPSCs before (blue) and after (red) application of leptin. Leptin increased the mean amplitude of sIPSCs at 2.5 mM glucose (2.5 mM, n =19 neurons; 5 mM, n =27 neurons; 10 mM, n =26 neurons). Scale bar, 20 pA, 20 ms. * P <0.05, *** P <0.001 versus control (paired t -test). All data are shown as mean±s.e.m. Full size image Table 1 Mean data of sIPSC and mIPSC frequency before and after addition of leptin. Full size table We then lowered external glucose levels from 10 to 5 mM. At 5 mM glucose, addition of leptin decreased GABAergic sIPSC frequency by 22% in one-fifth of POMC neurons ( n =6 out of 27 neurons; Fig. 1a,b and Table 1 ). Surprisingly, ~40% of POMC neurons responded to leptin with increased sIPSC frequency ( n =12 out of 27 neurons; Fig 1a,b and Table 1 ). The mean percent change in sIPSC frequency was 147.8±10.5% of control ( Fig. 1b and Table 1 ). When glucose levels were further lowered to 2.5 mM, the net effect of leptin on sIPSC frequency was stimulatory, which was in contrast with that observed at 10 mM glucose. In other words, leptin’s inhibitory effect on sIPSCs in POMC neurons was completely absent at 2.5 mM glucose ( n =0 out of 19 neurons examined). Addition of leptin raised sIPSC frequency in ~60% of POMC neurons ( n =12 out of 19 neurons; Fig. 1b and Table 1 ). The fraction of POMC neurons receiving enhanced GABA release was significantly higher at 2.5 mM than at 5 and 10 mM glucose levels ( Table 1 ). Importantly, differences in leptin’s action on sIPSC frequency were not because of changes in the baseline sIPSC activity as the baseline sIPSC frequency at different glucose levels was similar ([glucose] 2.5 mM, 2.4±0.4 Hz; 5 mM, 2.6±0.3 Hz; 10 mM, 2.6±0.5 Hz, n =19, 27 and 26 neurons, respectively). Given that leptin increases GABAergic inhibitory tone in a subset of POMC neurons, we sought to determine whether leptin-mediated enhancement of sIPSCs is able to inhibit POMC neuron activity. In current clamp configuration, addition of leptin (100 nM) induced a hyperpolarization in one-third of POMC neurons in the absence of the GABA A receptor antagonist at both 2.5 and 5 mM glucose ( Supplementary Fig. 1 and Supplementary Table 1 ). More importantly, leptin-induced hyperpolarization was completely abolished by the GABA A receptor antagonist ( Supplementary Fig. 1 and Supplementary Table 1 ), suggesting that enhanced GABAergic tone is sufficient to inhibit POMC neuron activity. Two distinct effects of leptin on GABAergic mIPSCs In the presence of tetrodotoxin (1 μM) to block the neuronal network activity, treatment with leptin increased the frequency of miniature IPSCs (mIPSCs) at 2.5 and 5 mM glucose ( Fig. 2a,b and Table 1 ). Only a few POMC neurons responded to leptin with reduced mIPSC frequency ( Fig. 2b and Table 1 ). 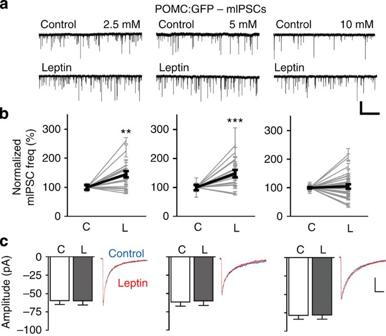Figure 2: Two distinct effects of leptin on mIPSCs. (a) Representative recording traces showing mIPSCs recorded from POMC neurons in the presence of tetrodotoxin (1 μM). Treatment with leptin (100 nM) increased mIPSC frequency in a subset of POMC neurons at 2.5, 5 and 10 mM glucose. HP=−70 mV. Scale bar, 100 pA, 10 s. (b) Graphs showing normalized frequency of mIPSCs from individual POMC neurons before and after treatment with leptin (bold line: total mean change in mIPSC frequency; 2.5 mM,n=20 neurons; 5 mM,n=21 neurons; 10 mM,n=31 neurons). C, control; L, leptin. (c) Pooled data showing mIPSC amplitude. Both superimposition of traces of sIPSCs before (blue) and after (red) application of leptin. Leptin did not change the mean amplitude of mIPSCs (2.5 mM,n=20 neurons; 5 mM,n=21 neurons; 10 mM,n=31 neurons). Scale bar, 20 pA, 20 ms. **P<0.01, ***P<0.001 versus control (pairedt-test). All data are shown as mean±s.e.m. Unlike the situation at 2.5 and 5 mM glucose, leptin either enhanced or reduced mIPSC frequency in POMC neurons at 10 mM glucose ( Fig 2a,b ). Leptin had no effect on mIPSC amplitude ( Fig. 2c ). There was no difference in the baseline mIPSC frequency under these conditions ([glucose] 2.5 mM, 1.1±0.2 Hz; 5 mM, 1.4±0.3 Hz; 10 mM, 1.4±0.2 Hz; n =20, 21 and 31 neurons, respectively). Figure 2: Two distinct effects of leptin on mIPSCs. ( a ) Representative recording traces showing mIPSCs recorded from POMC neurons in the presence of tetrodotoxin (1 μM). Treatment with leptin (100 nM) increased mIPSC frequency in a subset of POMC neurons at 2.5, 5 and 10 mM glucose. HP=−70 mV. Scale bar, 100 pA, 10 s. ( b ) Graphs showing normalized frequency of mIPSCs from individual POMC neurons before and after treatment with leptin (bold line: total mean change in mIPSC frequency; 2.5 mM, n =20 neurons; 5 mM, n =21 neurons; 10 mM, n =31 neurons). C, control; L, leptin. ( c ) Pooled data showing mIPSC amplitude. Both superimposition of traces of sIPSCs before (blue) and after (red) application of leptin. Leptin did not change the mean amplitude of mIPSCs (2.5 mM, n =20 neurons; 5 mM, n =21 neurons; 10 mM, n =31 neurons). Scale bar, 20 pA, 20 ms. ** P <0.01, *** P <0.001 versus control (paired t -test). All data are shown as mean±s.e.m. Full size image Activation of LepRs mediates synaptic upregulation We sought to determine the cellular mechanisms underlying leptin-mediated enhancement of IPSCs. Leptin receptors are expressed exclusively in somas and dendrites of POMC neurons [30] , and activation of LepRs on POMC neurons induces the release of the stimulatory peptide, α-MSH [27] . Cowley et al . [28] suggest the existence of an autoregulatory loop from opioid and melanocortin peptides and show the stimulatory effect of the MC3R agonist on GABA release. We thus examined whether activation of postsynaptic LepRs induces synaptic upregulation by using transgenic animals with selective deletion of LepRs in POMC neurons (that is, POMC-Cre:: LepR −/− mice [31] , [32] ). Leptin reduced mIPSC frequency without altering the mean amplitude in POMC-Cre:: LepR −/− mice at 5 mM glucose ( Fig. 3a,e ; mean amplitude, control, −63.9±6.0 pA; leptin, −62.4±6.6 pA; n =7 neurons). Importantly, no POMC neurons showed increased mIPSC frequency in response to leptin, which was in contrast with the net stimulatory effect of leptin on mIPSCs under the same experimental conditions (see Fig. 2a,b and Table 1 ). Hence, these results suggest that leptin’s stimulatory effect requires activation of postsynaptic rather than presynaptic LepRs on POMC neurons. 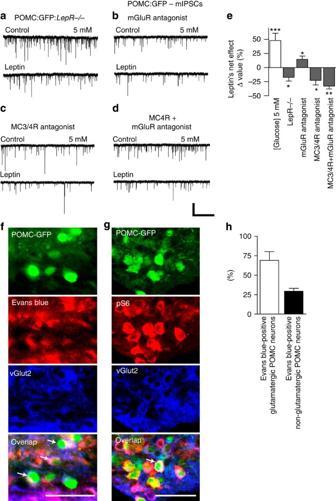Figure 3: Blockade of both MC3/4Rs and mGluRs inhibits leptin’s stimulatory effect. (a) Representative traces showing leptin’s effect on mIPSCs in POMC neurons from mice with selective deletion of leptin receptors in POMC neurons at 5 mM glucose levels. In contrast to the control group, leptin did not enhance the frequency of mIPSCs. HP=−70 mV. (b–d) Representative recording samples showing mIPSCs in the presence of the mGluR (MCPG;b), MC3/4R (SHU9119;c) antagonists or both (d) at 5 mM glucose. In the presence of the mGluR antagonist, leptin’s effect was significantly diminished compared with the control group. In the presence of the MC3/4R blocker alone or the MC3/4R and mGluR blockers, leptin no longer stimulated GABA release. Rather leptin had an inhibitory effect on mIPSCs. HP=−70 mV. Scale bar, 100 pA, 10 s. (e) Summary of leptin’s net effects on mIPSCs in mice lacking leptin receptors in POMC neurons and in the presence of the mGluR, MC3/4R antagonists or both. Pharmacological blockade of MC3/4Rs or mGluRs or both significantly attenuated or completely abolished leptin’s stimulatory effect on mIPSCs (LepR−/−,n=7 neurons; MCPG,n=19 neurons; SHU9119,n=9 neurons; MCPG+SHU9119,n=10 neurons). (f) Images of fluorescence microscopy showing the co-labelling of glutamatergic POMC neurons and Evans blue in the ARC. Glutamatergic neurons were found adjacent to and/or within the median eminence. More than two-third of glutamatergic POMC neurons were Evans blue-positive, suggesting that glutamatergic POMC neurons are directly exposed to blood glucose and leptin. (g) Images of fluorescence microscopy showing the co-expression of pS6 (red) and vGlut2 (blue) in a subset of POMC-GFP (green) neurons in the ARC of animal injected with leptin. Overall, 40% of glutamatergic POMC neurons were pS6-positive (n=9 out of 22 neurons). White arrow represents the POMC-GFP neuron co-expressing pS6 and vGlut2. Scale bar, 50 μm. (h) Percent of Evans blue-positive glutamatergic and nonglutamatergic POMC neurons. The majority of glutamatergic POMC neurons were Evans Blue-positive (n=5 animals). *P<0.05, **P<0.01, ***P<0.01 versus control (pairedt-test). All data are shown as mean±s.e.m. Figure 3: Blockade of both MC3/4Rs and mGluRs inhibits leptin’s stimulatory effect. ( a ) Representative traces showing leptin’s effect on mIPSCs in POMC neurons from mice with selective deletion of leptin receptors in POMC neurons at 5 mM glucose levels. In contrast to the control group, leptin did not enhance the frequency of mIPSCs. HP=−70 mV. ( b – d ) Representative recording samples showing mIPSCs in the presence of the mGluR (MCPG; b ), MC3/4R (SHU9119; c ) antagonists or both ( d ) at 5 mM glucose. In the presence of the mGluR antagonist, leptin’s effect was significantly diminished compared with the control group. In the presence of the MC3/4R blocker alone or the MC3/4R and mGluR blockers, leptin no longer stimulated GABA release. Rather leptin had an inhibitory effect on mIPSCs. HP=−70 mV. Scale bar, 100 pA, 10 s. ( e ) Summary of leptin’s net effects on mIPSCs in mice lacking leptin receptors in POMC neurons and in the presence of the mGluR, MC3/4R antagonists or both. Pharmacological blockade of MC3/4Rs or mGluRs or both significantly attenuated or completely abolished leptin’s stimulatory effect on mIPSCs ( LepR −/− , n =7 neurons; MCPG, n =19 neurons; SHU9119, n =9 neurons; MCPG+SHU9119, n =10 neurons). ( f ) Images of fluorescence microscopy showing the co-labelling of glutamatergic POMC neurons and Evans blue in the ARC. Glutamatergic neurons were found adjacent to and/or within the median eminence. More than two-third of glutamatergic POMC neurons were Evans blue-positive, suggesting that glutamatergic POMC neurons are directly exposed to blood glucose and leptin. ( g ) Images of fluorescence microscopy showing the co-expression of pS6 (red) and vGlut2 (blue) in a subset of POMC-GFP (green) neurons in the ARC of animal injected with leptin. Overall, 40% of glutamatergic POMC neurons were pS6-positive ( n =9 out of 22 neurons). White arrow represents the POMC-GFP neuron co-expressing pS6 and vGlut2. Scale bar, 50 μm. ( h ) Percent of Evans blue-positive glutamatergic and nonglutamatergic POMC neurons. The majority of glutamatergic POMC neurons were Evans Blue-positive ( n =5 animals). * P <0.05, ** P <0.01, *** P <0.01 versus control (paired t -test). All data are shown as mean±s.e.m. Full size image Leptin induces melanocortin and glutamate release As postsynaptic LepRs on POMC neurons are implicated in synaptic upregulation, it is plausible that leptin induces release of neuropeptides and neurotransmitters from POMC neurons, which upregulates GABA release. Hence, we investigated whether treatment with the MC3/4R (MTII, 100 nM) and mGlu receptor (mGluR; glutamate, 100 μM) agonists increases mIPSC frequency. The two reagents significantly increased mIPSC frequency ( Supplementary Fig. 2 ). These results suggest that activation of presynaptic MC3/4Rs and mGluRs on GABAergic axon terminals enhances GABA release. On the basis of these findings, we investigated whether leptin’s stimulatory effect on mIPSCs is mediated, in part, by presynaptic mGluRs. Treatment with the broad-spectrum mGluR antagonist MCPG (100 μM) significantly, but not completely, attenuated leptin’s stimulatory effect on mIPSC frequency at 5 mM glucose without changing mIPSC amplitude (mean amplitude, control, −54.6±4.3 pA; leptin, −55.8±5.4 pA; n =19 neurons). Thus, the total mean percent change in mIPSC frequency was significantly reduced compared with that observed without MCPG ( Fig. 3b,e ). We then examined whether pharmacological blockade of MC3/4Rs affects leptin’s stimulatory action on mIPSCs. Leptin’s stimulatory action on mIPSC frequency was completely absent in the presence of the MC3/4R antagonist SHU9119 (100 nM; Fig. 3c,e ; mean amplitude, control, −68.9±8.3 pA; leptin, −68.4±7.6 pA; n =9 neurons). However, leptin’s inhibitory effect on mIPSC frequency was still present. The total mean percent change in mIPSC frequency was 77.3±7.9% of control ( Fig. 3e ) We expanded our findings to determine whether co-application of both MC3/4R and mGluR antagonists inhibits leptin’s stimulatory effect. In the presence of SHU9119 and MCPG, leptin no longer facilitated mIPSC frequency ( Fig. 3d,e ; mIPSC amplitude, control, −66.2±9.7 pA; leptin, −65.2±10.1 pA; n =7 neurons). These findings suggest that neuropeptides and neurotransmitters from POMC neurons regulate the synaptic activity of neighbouring POMC neurons. To examine this possibility, we expressed a light-activated stimulatory protein channelrhodopsin exclusively in POMC neurons by crossbreeding the POMC-Cre with the channelrhodopsin (ChR2(H134R))-YFP animals. Bursts of light pulses (10 Hz) were applied for 1 s followed by a 3-s break that repeated five times. Blue light illumination of POMC neurons significantly increased sIPSC frequency ( Supplementary Fig. 3 ). A subset of glutamatergic POMC neurons respond to leptin Given that activation of LepRs in POMC neurons releases glutamate, we examined the expression of glutamatergic POMC neurons in the ARC. Glutamatergic POMC neurons were found adjacent to and/or within the median eminence, a circumventricular organ ( Supplementary Fig. 4 ). Thus, we investigated the anatomical relationship of glutamatergic POMC neurons with the brain–blood barrier (BBB) by using Evans blue, a commonly used fluorescent dye for assessing BBB permeability. This approach allows us to visualize glutamatergic POMC neurons that are in direct contact with the circulation. We found that a subset of POMC neurons were Evans blue-positive cells in the ARC. Surprisingly, the majority of glutamatergic POMC neurons were positive to Evans blue ( Fig. 3f,h ), while only one-fourth of nonglutamatergic POMC neurons were Evans blue-positive ( Fig. 3h ). Our results suggest that glutamatergic POMC neurons represent the predominant cell type situated outside and/or adjacent to the BBB in the ARC. Owing to this anatomical feature, glutamatergic POMC neurons appear to be directly exposed to blood-borne substances such as glucose and leptin. We then examined whether glutamatergic POMC neurons responded to leptin. We performed immunostaining with antibodies against vesicular glutamate transporter 2 (vGlut2) and phosphorylated S6 (pS6, an index of neuronal activity [33] ) following intraperitoneal (i.p.) injection of leptin. In fact, S6 is a structural component of the ribosome that is a distal target of PI3K signalling and is activated by phosphorylation [33] . Importantly, the JAK2–PI3K pathway plays a critical role in regulating POMC neuron activity independent of LepR/STAT3 signalling [34] . Hence, pS6 staining appears to be useful for measuring the leptin-mediated JAK2–PI3K pathway. Our data revealed that leptin induced the expression of pS6 in the ARC and ventromedial hypothalamus (VMH) of the hypothalamus ( Supplementary Fig. 4 ). Approximately one-fourth of POMC neurons from mice injected with leptin stained positive for pS6 ( n =241 out of 1,070 POMC-GFP (green fluorescent protein) neurons, Supplementary Fig. 4 ). Among POMC neurons, ~5% of POMC neurons were glutamatergic ( n =22 out of 477 neurons) and ~40% of glutamatergic POMC neurons were positive for pS6 ( n =9 out of 22 neurons, Fig. 3g ). TRPC channels mediate GABAergic enhancement It has been reported that calcium entry through TRPC channels triggers dendritic neurotransmitter release in the brain [35] . We investigated whether leptin-mediated TRPC channel opening induces the release of α-MSH and glutamate from POMC neurons. In the presence of the TRPC channel blocker 2-APB (100 μM), leptin failed to alter mIPSC frequency ( Fig. 4a,d and Table 2 ). As calcium influx through TRPC channels is important for dendritic release, we tested leptin in the absence of external calcium. Under these experimental conditions, most POMC neurons responded to leptin with a decrease in mIPSC frequency. The total mean percent change in mIPSC frequency was 83.6±5.3% of control ( Fig. 4b,d and Table 2 ). Moreover, the intracellular calcium release inhibitor dantrolene completely blocked leptin’s effect ( Supplementary Fig. 6 ). 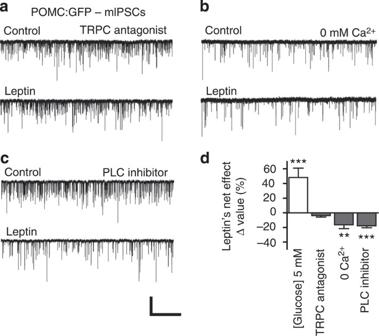Figure 4: TRPC channels mediate leptin’s stimulatory effect. (a) Representative recording samples showing mIPSCs recorded from POMC neurons in the presence of the TRPC channel blocker 2-APB. Leptin no longer modulated mIPSCs under these conditions. HP=−70 mV. (b) Sample traces showing mIPSCs recorded from POMC neurons following treatment with leptin in the absence of extracellular calcium. Leptin still reduced mIPSC frequency without extracellular calcium. (c) Representative recording samples showing mIPSCs recorded from POMC neurons in the presence of the PLC inhibitor U73122. Pharmacological blockade of PLC signalling abolished leptin’s stimulatory effect. Under these conditions, leptin remained effective in reducing GABA release. Scale bar, 100 pA, 10 s. (d) Summary plot showing leptin’s effect on mIPSC frequency following blockade of TRPC channel signalling (2-APB:n=9 neurons; 0 calcium:n=13 neurons; U73122:n=10 neurons). **P<0.01, ***P<0.001 versus control (pairedt-test). All data are shown as mean±s.e.m. Figure 4: TRPC channels mediate leptin’s stimulatory effect. ( a ) Representative recording samples showing mIPSCs recorded from POMC neurons in the presence of the TRPC channel blocker 2-APB. Leptin no longer modulated mIPSCs under these conditions. HP=−70 mV. ( b ) Sample traces showing mIPSCs recorded from POMC neurons following treatment with leptin in the absence of extracellular calcium. Leptin still reduced mIPSC frequency without extracellular calcium. ( c ) Representative recording samples showing mIPSCs recorded from POMC neurons in the presence of the PLC inhibitor U73122. Pharmacological blockade of PLC signalling abolished leptin’s stimulatory effect. Under these conditions, leptin remained effective in reducing GABA release. Scale bar, 100 pA, 10 s. ( d ) Summary plot showing leptin’s effect on mIPSC frequency following blockade of TRPC channel signalling (2-APB: n =9 neurons; 0 calcium: n =13 neurons; U73122: n =10 neurons). ** P <0.01, *** P <0.001 versus control (paired t -test). All data are shown as mean±s.e.m. Full size image Table 2 Summary of leptin’s effect on mIPSC and sIPSC frequency with drugs. Full size table As TRPC channels are activated by PLC stimulation in POMC neurons [15] , [36] , we blocked PLC with U73122 (10 μM). Leptin significantly reduced, but did not increase, mIPSC frequency with the PLC inhibitor U73122 (82.4±2.7% of control; Fig. 4c,d ). Hence, activation of TRPC channels by leptin contributes to GABAergic enhancement. Inhibition of AMPK by leptin decreases synaptic activity As leptin reduces mIPSC frequency following blockade of TRPC channels, we further sought to determine how leptin downregulates GABAergic synaptic activity. AMPK plays an important role in regulating neurotransmitter release in the ARC circuit [37] and is essential for glucose-sensing by POMC and AgRP neurons in the ARC [25] . Hence, we examined whether altered AMPK activity regulates GABAergic synaptic activity to POMC neurons as well. We found that the AMPK inhibitor dorsomorphin (10 μM) had an inhibitory effect on mIPSC frequency at 2.5 mM glucose at which leptin increased mIPSC frequency ( Fig. 5a,c ). In contrast, the AMPK activator A769662 (100 μM) increased mIPSC frequency by 40.4±11.8% at 10 mM glucose at which leptin reduced mIPSC frequency ( Fig. 5b,c ). 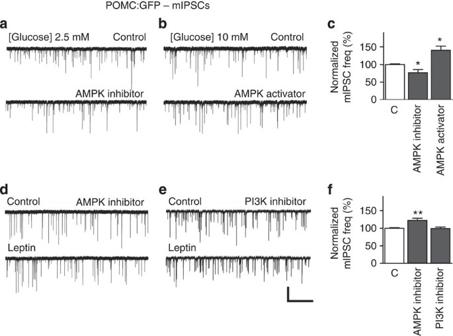Figure 5: Inhibition of presynaptic AMPK activity reduces mIPSC frequency. (a,b) Sample recording traces showing mIPSCs recorded from POMC neurons with the AMPK inhibitor dorsomorphin (a) and the AMPK activator A769662 (b). The AMPK inhibitor significantly decreased GABA release at 2.5 mM glucose (a), whereas the AMPK activator robustly increased mIPSC frequency at 10 mM glucose (b). The results suggest that presynaptic AMPK plays a major role in regulating GABA release. HP=−70 mV. Scale bar, 100 pA, 10 s. (c) Summary plot showing AMPK modulators’ effect on mIPSC frequency (dorsomorphin:n=6 neurons; A769662:n=7 neurons). C, control. (d,e) Representative recording samples showing leptin’s effect on mIPSCs recorded from POMC neurons in the presence of the AMPK inhibitor dorsomorphin and the PI3K inhibitor wortmannin at 5 mM glucose. Leptin increased mIPSC frequency in the presence of the AMPK inhibitor. The PI3K inhibitor completely abolished leptin’s action on mIPSCs. HP=−70 mV. Scale bar, 100 pA, 10 s. (f) Summary plot showing leptin’s effect on mIPSC frequency in the presence of the AMPK inhibitor and the PI3K inhibitor. As leptin no longer modulates mIPSCs in the presence of the PI3K inhibitor, both pre- and postsynaptic PI3K signalling is a key factor for leptin’s effect. However, presynaptic AMPK is involved in leptin-mediated reduction of GABA release (dorsomorphin:n=9 neurons; wortmannin:n=10 neurons). *P<0.05, **P<0.01 versus control (pairedt-test). All data are shown as mean±s.e.m. Figure 5: Inhibition of presynaptic AMPK activity reduces mIPSC frequency. ( a , b ) Sample recording traces showing mIPSCs recorded from POMC neurons with the AMPK inhibitor dorsomorphin ( a ) and the AMPK activator A769662 ( b ). The AMPK inhibitor significantly decreased GABA release at 2.5 mM glucose ( a ), whereas the AMPK activator robustly increased mIPSC frequency at 10 mM glucose ( b ). The results suggest that presynaptic AMPK plays a major role in regulating GABA release. HP=−70 mV. Scale bar, 100 pA, 10 s. ( c ) Summary plot showing AMPK modulators’ effect on mIPSC frequency (dorsomorphin: n =6 neurons; A769662: n =7 neurons). C, control. ( d , e ) Representative recording samples showing leptin’s effect on mIPSCs recorded from POMC neurons in the presence of the AMPK inhibitor dorsomorphin and the PI3K inhibitor wortmannin at 5 mM glucose. Leptin increased mIPSC frequency in the presence of the AMPK inhibitor. The PI3K inhibitor completely abolished leptin’s action on mIPSCs. HP=−70 mV. Scale bar, 100 pA, 10 s. ( f ) Summary plot showing leptin’s effect on mIPSC frequency in the presence of the AMPK inhibitor and the PI3K inhibitor. As leptin no longer modulates mIPSCs in the presence of the PI3K inhibitor, both pre- and postsynaptic PI3K signalling is a key factor for leptin’s effect. However, presynaptic AMPK is involved in leptin-mediated reduction of GABA release (dorsomorphin: n =9 neurons; wortmannin: n =10 neurons). * P <0.05, ** P <0.01 versus control (paired t -test). All data are shown as mean±s.e.m. Full size image On the basis of these findings, we examined whether leptin’s inhibitory effect on mIPSCs is because of reduced AMPK activity at 5 mM glucose. Leptin no longer depressed, but clearly enhanced, mIPSC frequency in the presence of the AMPK inhibitor dorsomorphin ( Fig. 5d,f ). The total mean percent change in mIPSC frequency was 122.1±6.5% of control ( Fig. 5f ). These results suggest that suppression of AMPK activity in presynaptic GABA terminals reduces GABA release. In addition, we also investigated whether blockade of K ATP channels influences leptin’s action on GABA release as K ATP channels appears to be a downstream target of leptin [38] . However, inhibition of K ATP channels did not affect leptin’s action on mIPSCs ( Supplementary Fig. 5 ). Interestingly, the leptin-mediated JAK2–PI3K pathway regulates both AMPK and PLC signalling pathways [15] , [23] . It is thus possible that blockade of PI3K abolishes leptin’s stimulatory and inhibitory effects on mIPSCs. Indeed, we found that leptin had no effect on mIPSCs in the presence of the PI3K inhibitor wortmannin at 5 mM glucose (100 nM; Fig. 5e,f ). Furthermore, blockade of JAK2 completely abolished the effects of leptin on mIPSCs ( Supplementary Fig. 7 ). To summarize, inhibition of presynaptic AMPK activity by leptin reduces, whereas activation of postsynaptic PLC in POMC neurons enhances GABA release. Both effects are mediated by the JAK2–PI3K signalling pathway. High-fat feeding disrupts leptin’s action on sIPSCs It has been reported that the baseline AMPK activity in the hypothalamus is downregulated in animals fed a high-fat diet (HFD). More importantly, leptin fails to further reduce AMPK activity in diet-induced obesity (DIO) mice [24] . We tested the hypothesis that high-fat feeding preferentially suppresses leptin’s inhibitory action on GABA release to POMC neurons. We performed experiments on POMC neurons from animals fed a HFD for 3 weeks. Under these conditions, treatment with leptin facilitated, but did not depress, GABAergic sIPSCs at 10 mM glucose at which leptin had an inhibitory effect on sIPSCs in the control group ( Fig. 6a,e ). These results were in contrast to those observed in animals fed a normal chow diet (NCD; Fig. 6e ). As reduced AMPK activity can result in this alteration, we further examined whether pharmacological activation of AMPK is able to reverse enhanced GABAergic sIPSCs. Incubation of hypothalamic slices with the AMPK activator for 1–2 h completely reversed leptin’s stimulatory effect at 10 mM glucose ( Fig. 6b,e ). We further determined whether leptin’s stimulatory effect is because of activation of MC3/4Rs and mGluRs as well. In the presence of the MC3/4R and mGluR antagonists, leptin no longer increased sIPSC frequency; however, leptin’s inhibitory effect was still present in animals on a HFD ( Fig. 6c–e ). 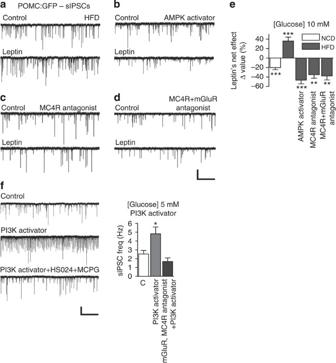Figure 6: High-fat feeding alters leptin’s action on sIPSCs. (a,b) Representative sample traces showing sIPSCs recorded from POMC neurons in animals fed HFD for 3 weeks. In contrast to the control group, leptin significantly increased sIPSC frequency at 10 mM glucose (a). Leptin reduced sIPSC frequency, suggesting that the AMPK activator completely reverses leptin’s action on sIPSCs. HP=−70 mV. (c,d). Sample recording traces showing sIPSCs recorded from POMC neurons in animals on HFD in the presence of the MC3/4R antagonist alone or the MC3/4R and mGluR antagonists. Leptin had an inhibitory effect on sIPSCs under these conditions. HP=−70 mV. Scale bar, 100 pA, 10 s. (e) Summary plot showing leptin’s net effect on sIPSCs recorded from POMC neurons at 10 mM glucose in animals fed NCD and HFD. Leptin had opposing effects on sIPSCs at 10 mM glucose in animals fed NCD and HFD (n=14 neurons). Leptin’s stimulatory effect was completely inhibited by the AMPK activator and MC3/4R antagonist (A769662,n=7 neurons; SHU9119,n=8 neurons; MCPG+SHU9119,n=8 neurons). NCD, normal chow diet; HFD, high-fat diet. (f) Sample recording traces (left) and summary plot (right) of sIPSCs recorded from POMC neurons in animals microinjected with the PI3K activator or the activator plus the MC3/4R and mGluR antagonists. Injection of the PI3K activator strongly increased sIPSC frequency, which was completely blocked by the MC3/4R and mGluR antagonists (n=24 and 16 neurons, respectively). Scale bar, 100 pA, 10 s. *P<0.05, **P<0.01, ***P<0.001 versus control (pairedt-test). All data are shown as mean±s.e.m. Figure 6: High-fat feeding alters leptin’s action on sIPSCs. ( a , b ) Representative sample traces showing sIPSCs recorded from POMC neurons in animals fed HFD for 3 weeks. In contrast to the control group, leptin significantly increased sIPSC frequency at 10 mM glucose ( a ). Leptin reduced sIPSC frequency, suggesting that the AMPK activator completely reverses leptin’s action on sIPSCs. HP=−70 mV. ( c , d ). Sample recording traces showing sIPSCs recorded from POMC neurons in animals on HFD in the presence of the MC3/4R antagonist alone or the MC3/4R and mGluR antagonists. Leptin had an inhibitory effect on sIPSCs under these conditions. HP=−70 mV. Scale bar, 100 pA, 10 s. ( e ) Summary plot showing leptin’s net effect on sIPSCs recorded from POMC neurons at 10 mM glucose in animals fed NCD and HFD. Leptin had opposing effects on sIPSCs at 10 mM glucose in animals fed NCD and HFD ( n =14 neurons). Leptin’s stimulatory effect was completely inhibited by the AMPK activator and MC3/4R antagonist (A769662, n =7 neurons; SHU9119, n =8 neurons; MCPG+SHU9119, n =8 neurons). NCD, normal chow diet; HFD, high-fat diet. ( f ) Sample recording traces (left) and summary plot (right) of sIPSCs recorded from POMC neurons in animals microinjected with the PI3K activator or the activator plus the MC3/4R and mGluR antagonists. Injection of the PI3K activator strongly increased sIPSC frequency, which was completely blocked by the MC3/4R and mGluR antagonists ( n =24 and 16 neurons, respectively). Scale bar, 100 pA, 10 s. * P <0.05, ** P <0.01, *** P <0.001 versus control (paired t -test). All data are shown as mean±s.e.m. Full size image As POMC neurons in animals fed a HFD respond to leptin with increased GABA release, we sought to determine whether short-term activation of PI3K upregulates inhibitory tone to POMC neurons. Microinjection of the PI3K activator (5 mg ml −1 ) into the mediobasal hypothalamus (MBH) 12 h before recording sessions significantly increased the baseline GABAergic activity from 2.5±0.4 to 4.8±0.8 Hz ( Fig. 6f ). More importantly, this effect was completely abolished by co-injection of the MC3/4R and mGluR antagonists ( Fig 6f ). These findings suggest that upregulation of the PI3K pathway provokes synaptic feedback inhibition of POMC neurons. High-fat feeding upregulates JAK2–PI3K signalling We expanded our findings to determine the physiological consequences of these synaptic alterations in POMC neurons at the whole-body level. We measured body weight, calorie intake, plasma glucose, leptin and insulin levels after 3 weeks on a HFD. Body weight and calorie intake in animals fed a HFD were no different from the control (body weight, NCD 19.9±0.6 g, HFD 19.8±0.5 g; calorie intake, NCD, 13.5±0.5 kcal g −1 , HFD, 12.6±0.3 kcal g −1 ; Fig. 7a,b ). However, the ratio of fat tissue to lean mass was significantly higher in animals fed a HFD than in animals on NCD (0.3±0.02 versus 0.4±0.02; Fig. 7c ). This was associated with elevated blood glucose and leptin levels ( Fig. 7d,e ). 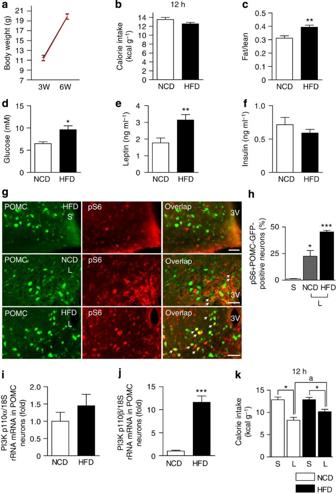Figure 7: High-fat feeding upregulates JAK2–PI3K signalling. (a,b) Body weight and calorie intake of animals fed NCD (control,n=15 animals) and HFD (n=18 animals) after 3 weeks. There was no difference between control (NCD) and HFD animals. NCD, normal chow diet; HFD, high-fat diet. (c) Ratio of fat tissue to lean mass for control (n=10 animals) and HFD (n=14 animals) groups. High-fat feeding significantly increased the ratio of fat tissue to lean mass. (d–f) Plasma glucose, leptin and insulin levels after 3 weeks on HFD. Plasma glucose and leptin levels were significantly elevated in animals fed HFD (glucose,n=8 animals; leptin,n=14 animals) compared with control (glucose,n=7 animals;n=16 animals). However, insulin levels were similar in both groups. (g,h) Images of fluorescence microscopy showing the co-expression of pS6 (red) and POMC neurons (green) in the ARC of animal injected with leptin (g). Summary plot (h) showing the percent of pS6-positive POMC neurons in animals fed a NCD (n=9 animals) and a HFD (n=8 animals). There was a significant increase in the number of pS6-positive POMC neurons in animals fed HFD. Scale bar, 50 μm. S, saline; L, leptin. (i,j) PI3K p110α (i) and p110β (j) mRNA expression in POMC neurons. The dietary intervention significantly increased the expression of p110β, but not p110α, mRNAs in POMC neurons (p110α, NCD,n=6 neurons, HFD,n=5 neurons; p110β, NCD,n=6 neurons, HFD,n=9 neurons). (k) Calorie intake for control and HFD groups after microinjection of leptin into the MBH. High-fat feeding significantly diminished leptin’s anorexigenic effects (NCD,n=14 animals, HFD,n=18 animals). *P<0.05, **P<0.01, ***P<0.001 versus control (unpairedt-test);aP<0.05 versus NCD+leptin (unpairedt-test). All data are shown as mean±s.e.m. Figure 7: High-fat feeding upregulates JAK2–PI3K signalling. ( a , b ) Body weight and calorie intake of animals fed NCD (control, n =15 animals) and HFD ( n =18 animals) after 3 weeks. There was no difference between control (NCD) and HFD animals. NCD, normal chow diet; HFD, high-fat diet. ( c ) Ratio of fat tissue to lean mass for control ( n =10 animals) and HFD ( n =14 animals) groups. High-fat feeding significantly increased the ratio of fat tissue to lean mass. ( d – f ) Plasma glucose, leptin and insulin levels after 3 weeks on HFD. Plasma glucose and leptin levels were significantly elevated in animals fed HFD (glucose, n =8 animals; leptin, n =14 animals) compared with control (glucose, n =7 animals; n =16 animals). However, insulin levels were similar in both groups. ( g , h ) Images of fluorescence microscopy showing the co-expression of pS6 (red) and POMC neurons (green) in the ARC of animal injected with leptin ( g ). Summary plot ( h ) showing the percent of pS6-positive POMC neurons in animals fed a NCD ( n =9 animals) and a HFD ( n =8 animals). There was a significant increase in the number of pS6-positive POMC neurons in animals fed HFD. Scale bar, 50 μm. S, saline; L, leptin. ( i , j ) PI3K p110α ( i ) and p110β ( j ) mRNA expression in POMC neurons. The dietary intervention significantly increased the expression of p110β, but not p110α, mRNAs in POMC neurons (p110α, NCD, n =6 neurons, HFD, n =5 neurons; p110β, NCD, n =6 neurons, HFD, n =9 neurons). ( k ) Calorie intake for control and HFD groups after microinjection of leptin into the MBH. High-fat feeding significantly diminished leptin’s anorexigenic effects (NCD, n =14 animals, HFD, n =18 animals). * P <0.05, ** P <0.01, *** P <0.001 versus control (unpaired t -test); a P <0.05 versus NCD+leptin (unpaired t -test). All data are shown as mean±s.e.m. Full size image In order to determine whether high-fat feeding affects LepR signalling in POMC neurons, we measured both pS6 and pSTAT3 expression in POMC neurons from animals on a HFD following i.p. injection of leptin. The percent of pS6 expression in POMC neurons was significantly higher in the HFD group than in the control NCD group ( Fig. 7g,h ), although there was no change in pSTAT3-positive POMC cells following high-fat feeding ( Supplementary Fig. 4d ). We further measured PI3K (both p110α and p110β isoforms) mRNA levels in individual POMC neurons with single-cell real-time quantitative reverse transcription–PCR (qRT–PCR). High-fat feeding robustly elevated the expression of p110β, but not p110α, mRNAs in POMC neurons from animals fed a HFD ( Fig. 7i,j ). We also noted that the fraction of AMPK α2-expressing POMC neurons was decreased in animals on high-fat feeding ( Supplementary Fig. 8 ) We then determined whether increased PI3K levels in POMC neurons in the HFD group influenced leptin’s effects on calorie intake. Leptin (50 ng per 0.5 μl) was directly infused into the MBH. The NCD group consumed significantly less than the HFD group did after microinjection of leptin, although leptin still reduced food intake in animals fed a HFD ( Fig. 7k ). Therefore, leptin-mediated upregulation of GABAergic transmission would play a role in the regulation of ingestive behaviour ( Fig. 8 ). 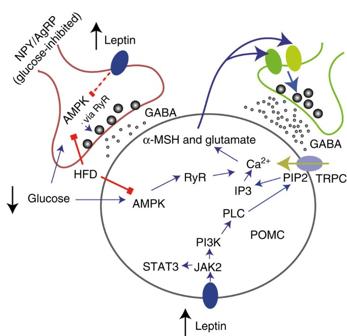Figure 8: Schematic illustration of the proposed model. Alterations in glucose levels regulate AMPK activity in the ARC circuit. Inhibition by leptin of AMPK in presynaptic GABAergic axon terminals reduces GABA release to POMC cells. In contrast, leptin receptor activation on POMC neurons stimulates the JAK2–PI3K–PLC pathway, resulting in opening of TRPC channels and probably inositol 1,4,5-trisphosphate receptors as well. Increased Ca2+concentrations trigger the release of melanocortin and glutamate from glutamatergic POMC neurons. Short-term exposure to a high-fat diet upregulates PI3K activity specifically in POMC neurons. Under these conditions, leptin no longer reduces GABA release from presynaptic GABAergic neurons. However, the JAK2–PI3K–PLC pathway by leptin in POMC neurons remains effectively transmitted, thereby enhancing GABAergic inhibitory tone to POMC neurons. This feedback inhibition of POMC neurons in animals on high-fat feeding may play a role in the regulation of overall energy balance. Figure 8: Schematic illustration of the proposed model. Alterations in glucose levels regulate AMPK activity in the ARC circuit. Inhibition by leptin of AMPK in presynaptic GABAergic axon terminals reduces GABA release to POMC cells. In contrast, leptin receptor activation on POMC neurons stimulates the JAK2–PI3K–PLC pathway, resulting in opening of TRPC channels and probably inositol 1,4,5-trisphosphate receptors as well. Increased Ca 2+ concentrations trigger the release of melanocortin and glutamate from glutamatergic POMC neurons. Short-term exposure to a high-fat diet upregulates PI3K activity specifically in POMC neurons. Under these conditions, leptin no longer reduces GABA release from presynaptic GABAergic neurons. However, the JAK2–PI3K–PLC pathway by leptin in POMC neurons remains effectively transmitted, thereby enhancing GABAergic inhibitory tone to POMC neurons. This feedback inhibition of POMC neurons in animals on high-fat feeding may play a role in the regulation of overall energy balance. Full size image In this study, we outlined the cellular mechanisms underlying the effect of leptin on GABA release. We found that inhibition of AMPK by leptin in presynaptic terminals decreased GABA release at 10 mM glucose. However, activation of somatic LepRs on POMC neurons stimulated PLC activity, resulting in opening of TRPC channels. Ca 2+ -permeable TRPC channels generated changes in the intracellular calcium concentration, thereby causing the release of α-MSH and glutamate from glutamatergic POMC neurons at 2.5 mM glucose. Activation of presynaptic MC3/4 and mGlu receptors elevated GABA release. Hence, GABAergic synapses to POMC neurons differentially responded to leptin at different levels of glucose. AMPK appears to be responsible for the interplay between glucose and leptin signalling. Furthermore, high-fat feeding blunted AMPK-dependent presynaptic inhibition, whereas PLC-mediated GABAergic feedback inhibition remained responsive to leptin. Therefore, in mice fed a HFD, leptin enhanced rather than reduced GABA release to POMC neurons. This unexpected finding appears to be paradox as inhibition of POMC neurons would increase food intake. Previous studies describe direct and indirect regulation of POMC neurons by activation of MC3/4Rs (ref. 39 ) and/or μ-opioid receptors [28] , [40] . Furthermore, recent studies illustrate that hypothalamic POMC neurons have distinct neurotransmitter phenotypes [29] , [41] , [42] . Less than half of POMC neurons are GABAergic, while a subset of non-GABAergic POMC neurons is glutamatergic [29] , [42] , [43] . Moreover, POMC is cleaved enzymatically into diverse peptides, including α-MSH and β-endorphin. POMC neurons thus produce and release two distinct peptides, α-MSH and β-endorphin, which have opposing actions on ingestive behaviour; α-MSH is anorexigenic (appetite-suppressing), whereas β-endorphin appears to be orexigenic (appetite-stimulating) [44] , [45] , [46] . Recent studies also demonstrate that selective stimulation of POMC neurons appears to induce the release of either opioid alone or melanocortin alone at the cellular and whole-body levels since the effects of optogenetic stimulation of POMC neurons are blocked by either the opioid or the melanocortin receptor antagonists, respectively [37] , [47] . POMC neurons are thus likely to be phenotypically and perhaps functionally heterogeneous unlike AgRP neurons, which are all GABAergic [29] . This heterogeneity of POMC neurons raises fundamental questions as to their precise identity, distribution as well as function. Although POMC neurons sense and respond to both glucose and leptin [26] , [28] , [48] , the role of glucose-sensing by POMC neurons on leptin’s action has not been well studied. Both glucose and leptin induce α-MSH release from POMC neurons [26] , [27] . Hence, it is important to know how POMC neurons integrate these two signal molecules at the synaptic level and whether this integration influences POMC neuronal activity, resulting in changes in feeding behaviour and ultimately body weight. The cellular mechanisms that mediate glucose-sensing by POMC neurons have been well documented. For instance, opening of K ATP channels by lowering glucose levels decreases POMC neuron activity [26] . In addition, stimulation of AMPK by reducing glucose levels is responsible for glucose-sensing as mice lacking the AMPK α2 in POMC neurons do not respond to alterations in glucose levels [25] . Of particular interest is that AMPK activity is altered by leptin as well [22] , [23] . Thus, it seems likely that POMC neurons integrate nutrients and adiposity signals through alteration in AMPK activity. Activation of the LepR stimulates diverse signalling pathways in POMC neurons. For instance, activation of LepRs in POMC neurons regulates POMC mRNAs via the JAK2–STAT3 signalling [21] . In addition, leptin stimulates the JAK2–PI3K pathway in POMC neurons. In fact, mice lacking STAT3 in POMC neurons still show leptin-induced hypophagia [49] and GABAergic inputs to POMC neurons remain responsive to leptin in animals expressing LepRb defective for STAT3 signalling [34] . Recent studies further highlight the contribution of the JAK2–PI3K pathway to the regulation of POMC neuronal activity. First, indirect continuous stimulation of PI3K activity through inhibition of Pten in POMC neurons affects leptin’s electric effect [16] . Of particular interest is that mice lacking Pten in POMC neurons exhibit a marked hyperpolarization that is associated with a reduction in the baseline firing rate [16] . We also observed that microinjection of the PI3K activator enhanced inhibitory tone, further supporting that increased PI3K activity reduces POMC neuron activity. Second, POMC neurons in mice with genetically disrupted PI3K signalling do not respond to leptin. Third, leptin has no effect on POMC neurons in mice lacking the p110β isoform of PI3K (ref. 18 ). Importantly, short-term exposure to a HFD increased plasma leptin levels as well as p100β expression in POMC neurons. Fourth, leptin stimulates TRPC channels via the JAK2–PI3K–PLC pathway [15] . Finally, our current data showed the contribution of PI3K signalling to leptin’s electrophysiological action as blockade of JAK2 or PI3K completely blunted leptin’s presynaptic as well as postsynaptic effects. Hence, leptin-induced JAK2–PI3K pathway plays a key role in regulating POMC neuron function. Despite the renowned effects of leptin on GABA release to POMC neurons [28] , [29] , the cellular mechanisms remain elusive. It has been described that stimulation of AMPK by fasting or ghrelin increases the release of neurotransmitters to AgRP neurons via ryanodine receptors [37] . In line with these findings, we showed that alterations in AMPK activity in presynaptic terminals modulated GABA release to POMC neurons. More importantly, inhibition of AMPK completely abolished leptin’s inhibitory effect on GABA release. We should emphasize that, although reduced GABA release was independent of extracellular calcium, leptin failed to reduce GABA release when intracellular calcium release was blocked with the ryanodine receptor inhibitor dantrolene. We thus propose that inhibition of AMPK in GABAergic terminals reduces calcium release from ryanodine receptors, thereby decreasing GABA release to POMC neurons. Hence, our results provide detailed insights into how leptin regulates GABA release in the ARC neural circuit. In contrast to leptin’s inhibitory effect of GABA release, leptin’s excitatory effect was postsynaptic in origin. In other words, activation of LepRs in POMC neurons enhanced GABA release because deletion of LepRs in POMC neurons completely blunted the effect. Moreover, the release of α-MSH and glutamate is a causal factor in enhancing GABA release. Indeed, POMC neurons receive GABAergic inputs regulated by MC3/4Rs, suggesting that melanocortin peptides have an autoinhibitory effect on POMC neuronal activity [28] . We found that TRPC channels located in POMC neurons contributed to the upregulation of GABAergic transmission. In fact, it has been reported that calcium entry through TRPC channels controls dendritic neurotransmitter release in the thalamus [35] . Moreover, a series of experiments (that is, 0 mM [calcium] ext , the TRPC blocker and PLC inhibitor) support the contribution of TRPC channels to the release of glutamate and melanocortin peptides. We also note that the release of melanocortin and glutamate was still present without neuronal activity (that is, under tetrodotoxin treatment). A recent immunohistochemical study demonstrates the expression of LepRs exclusively in somas and dendrites, but not in axon terminals, of POMC neurons [30] . It is thus plausible that activation of somatic and/or dendritic LepRs stimulates TRPC channels on POMC neurons and subsequently causes calcium entry into the cytoplasm, thereby inducing neurotransmitter release from somas/dendrites of POMC neurons. Why and how does leptin induces the release of melanocortin and glutamate especially at low levels of glucose? Among TRPC channels, TRPC1, 4 and 5, which are highly expressed in POMC neurons [15] , are positively regulated by intracellular calcium [50] . Recent work described in ref. 37 demonstrates that activation of AMPK stimulates ryanodine receptors that can generate increased calcium levels in axon terminals. Hence, it is also plausible that lowering glucose levels stimulates AMPK and ryanodine receptors in POMC neurons. Sustained rise in cytosolic calcium levels from intracellular calcium pools would facilitate channel activity. As a result, calcium influx through TRPC channels by leptin would be more robust at low than at high glucose levels. In addition, this would be further enhanced by production of (IP3) through the PLC pathway. Therefore, we propose that alterations in AMPK activity require leptin’s inhibitory and excitatory effects on GABA release. AMPK plays a key role in integrating nutrients and adiposity signals at GABAergic synapses to POMC neurons. Central leptin resistance developed after long-term exposure to a HFD (>15 weeks) [27] , [51] , [52] , [53] . Indeed, we showed that the JAK2–PI3K signalling pathway was intact in POMC neurons, although animals fed a HFD for 3 weeks showed elevated leptin levels. In particular, we demonstrated that high-fat feeding significantly increased the expression of p110β mRNA levels specifically in POMC neurons. Moreover, this was associated with reduced AMPK α2 mRNA levels in POMC neurons. Although it has been shown that high-fat feeding lowers the basal AMPK activity and abolishes leptin’s ability to reduce AMPK activity in the hypothalamus [24] , our present study further suggests that short-term high-fat feeding alters AMPK as well as PI3K activity in POMC neurons. At GABAergic synapses to POMC neurons, high-fat feeding diminishes leptin’s inhibitory effect on GABA release via downregulation of presynaptic AMPK activity. In contrast, intracellular signals via the PLC pathway are still effectively transmitted, thereby enhancing GABAergic inhibitory tone on POMC neurons at the postsynaptic level. Leptin-mediated upregulation of GABAergic transmission would result in inhibition of POMC neurons. Hence, this feedback inhibition of POMC neurons would play a role in the regulation of ingestive behaviour. Animals All mouse care and experimental procedures were approved by the Institutional Animal Care Research Advisory Committee of the Albert Einstein College of Medicine. Mice used in these experiments included POMC-CRE, Z/EG, LepR flox/flox (POMC-Cre:: LepR −/− (ref. 31 )) and POMC-GFP (The Jackson Laboratory) mice. Male and female mice of mixed C57BL/6, FVB and 129 strain background were used at the postnatal age of 28–35 days for all experiments. Slice preparation Transverse brain slices were prepared from transgenic mice. Animals were anaesthetized with isoflurane. After decapitation, the brain was transferred into a sucrose-based solution bubbled with 95% O 2 /5% CO 2 and maintained at ~3 °C. This solution contained the following (in mM): 248 sucrose, 2 KCl, 1 MgCl 2 , 1.25 KH 2 PO 4 , 26 NaHCO 3 , 1 sodium pyruvate and 10 glucose. Transverse coronal brain slices (200 μm) were prepared using a vibratome. Slices were equilibrated with an oxygenated artificial cerebrospinal fluid (aCSF) for >1 h at 32 °C before being transferred to the recording chamber. The slices were continuously superfused with aCSF at a rate of 1.5 ml min −1 containing the following (in mM): 113 NaCl, 3 KCl, 1 NaH 2 PO 4 , 26 NaHCO 3 , 2.5 CaCl 2 , 1 MgCl 2 and 2.5, 5 or 10 glucose in 95% O 2 /5% CO 2 . Electrophysiological recordings Brain slices were placed on the stage of an upright, infrared-differential interference contrast microscope (Olympus BX50WI) mounted on a Gibraltar X-Y table (Burleigh) and visualized with a × 40 water-immersion objective using infrared microscopy (DAGE MTI camera). The internal solution contained the following (in mM): 130 CsCl (or KCl), 5 CaCl 2 , 10 EGTA, 10 HEPES, 2 MgATP, 0.5 Na 2 GTP and 5 phosphocreatine. All recordings were made at 30±2 °C. GABAergic currents were isolated by addition of 6-Cyano-7-nitroquinoxaline-2,3-dione (10 μM) and D -amino-phosphovaleric acid (50 μM). Membrane currents were recorded with a Multiclamp 700B in the whole-cell configuration. Electrophysiological signals were low-pass-filtered at 2–5 kHz, stored on a PC and analysed offline with the pClamp 10 software (Molecular devices, CA) and the Mini Analysis software version 6 (Synaptosoft Inc). For each recording, the averaged IPSC event number and membrane potential from every 30-s epoch were taken as one data point. A total of 10 data points before and after application of leptin was compared using the unpaired t -test. If the P value was less than 0.05, cells were considered to be leptin-responsive. In some experiments, extracellular calcium ions were removed from aCSF (that is, [Calcium] ext 0 mM) and 1 mM EGTA was added. To examine whether the responses to leptin are regulated by dietary history, two groups of animals were fed a standard diet (with 60% calories provided by carbohydrates, 20% by protein and 5% by fat) or a high-fat diet (with 20% calories by carbohydrate, 20% by protein and 60% by fat) for 3 weeks starting from the postnatal age of 21 days. The PI3K activator (5 mg ml −1 ) alone or with HS024 (0.13 mg ml −1 ) and MCPG (20 mg ml −1 ) was microinjected into the mediobasal hypothalamus of the POMC-GFP mice in some experiments as noted. Stereotaxic surgery and leptin infusion Mice were maintained under isoflurane anaesthesia and placed in a stereotaxic apparatus (David Kopf Instruments). Under aseptic conditions, sterile custom guide cannulas (Plastics One Inc.) were stereotaxically implanted into the MBH (anteroposterior (AP), −1.2 mm; mediolateral (ML), 0; dorsoventral (DV), −5.5 mm). Animals were allowed at least 3 days to recover from surgery. To measure food intake, animals were separated individually in single cage for 5 days and fasted for 6 h (from 1300 to 1900 h) before leptin infusion. Leptin (50 ng per 0.5 μl) was infused directly into the MBH at 1800 h. Body composition and energy balance measurements Total fat and lean mass of mice were analysed using the EchoMRI system (Echo Medical systems). Food intake per mouse was measured 12-h post-icv injection of leptin in animals fed a NCD and a HFD. Body weights and food intake were measured on a scale with 0.1-g accuracy. Blood glucose and plasma leptin/insulin assay Blood glucose levels were measured every 4 h for 24 h using a Bayer Ascensia Elite glucose meter. Blood samples were collected into tubes with lithium heparin (VWR international, LLC) and centrifuged at 3,000 r.p.m. for 15 min to collect plasma. Plasma leptin and insulin levels were quantified using the ELISA assay (Mouse leptin ELISA kit, EMD Millipore; Mouse insulin ELISA kit, ALPCO Corp.) by the Albert Einstein College of medicine hormone assay core. Immunostaining Animals at the postnatal age of 6 weeks were treated with either 1-mg kg −1 -body weight leptin or saline for 1 h. Mice were anaesthetized with isoflurane and perfused transcardially with 10 ml of cold 1 × PBS followed by 25 ml of 4% paraformaldehyde (PFA). Brains were immediately removed, and postfixed in 4% PFA at 4 °C overnight. The complete rostral to caudal extension of the ARC was cut in 40-μm coronal sections with a vibratome. Sections were blocked with 5% bovine serum albumin (Sigma-Aldrich) for 2 h at room temperature, and then incubated with anti-pS6 (Cell Signaling, 2215S), anti-pSTAT3 (Cell Signaling, 9145S), anti-vGlut2 (Millipore, MAB5504) and anti-GFP (Millipore, 06-896) antibodies (1:1,000; 1:500; 1:500; 1:500) diluted in 0.5% Triton X-100 in PBS for 2 days at 4 °C. For vGlut2 staining, colchicine (1 μl of 10 mg ml −1 ) was injected into the lateral ventricle of animals 1 day before being killed. Sections were washed three times in PBS, and then incubated in 1:500 diluted Alexa Fluor 405 anti-mouse IgG (Life Technologies, A31553), Alexa Fluor 488 anti-chicken IgG (Millipore, AP194F) and Alexa Fluor 568 anti-rabbit IgG (Life Technologies, A11008) in 0.5% Triton X-100 in PBS for 3 h at room temperature. Tissues were then washed three times in PBS, dried and mounted with VECTASHIELD mounting media (Vector Labs). Images were acquired using a Leica scanning confocal microscope (Heidelberg, Germany). Single-Cell qRT–PCR analysis Single-cell samples were collected from brain slice preparations via aspiration into the patch pipette. The initial reverse transcription (RT) reaction was conducted after pressure ejection of the single-cell samples into a microcentrifuge tube with the REPLI-g WTA single cell kit (Qiagen). Samples were incubated in a total volume of 2.5 μl at 24 °C for 5 min and cooled to 4 °C. Samples were then incubated for 10 min at 42 °C with 0.5 μl gDNA wipeout buffer before addition of 1.75 μl RT mix to synthesize first strand cDNA (RT mix: 0.25 μl oligodT primer, 1 μl RT buffer, 0.25 μl random primer and 0.25 μl RT enzyme mix). The tubes were incubated at 42 °C for 1 h, and at 95 °C for 3 min. The tubes then were incubated at 24 °C for 30 min with 2.5 μl ligation mix (2 μl ligase buffer and 0.5 μl ligase Mix). The reaction was stopped by incubating at 95 °C for 5 min. Samples were incubated at 30 °C for 2 h after adding the amplification mix (7.25 μl buffer and 0.25 μl REPLI-g SensiPhi DNA polymerase) and at 65 °C for 5 min. The concentration of purified single-cell whole cDNA was measured using a NanoDrop 8000 spectrophotometer (Thermo Scientific). Single-cell real-time qPCR was performed in sealed 96-well plates with SYBR Green I master Mix by using a Light Cycler 480 instrument (Roche Applied Science). The 18S ribosomal RNA was used as an internal positive control for normalization of each sample. qPCR reactions were prepared in a final volume of 20 μl containing 2 μl of single-cell whole cDNA, and 10 μl of SYBR Green master mix in the presence of primers at 0.5 μM. The primers used for qPCR were as follows for the PI3K 110α, PI3K 110β, AMPK α2 and 18S genes. PI3K 110α -F, 5′- GTGAACTGGATGGCTCACAC -3′; PI3K 110α -R, 5′- ATGGAAAGGAAACGAACAGG -3′; PI3K 110β -F, 5′- GCATTTCTTCCAGCTCATCA -3′; PI3K 110β-R , 5′- ATCAGACCATCAGGAAAGCC -3′; AMPK α2 -F, 5′- CTCCCAGGGTGAAGTCTCAT -3′; AMPK α2 -R, 5′- CTGAAGGACAAGTTGCCAGA -3′; 18S-F, 5′-CTCAACACGGGAAACCTCAC-3′; 18S-R, 5′-CGCTCCACCAACTAAGAACG-3′. A standard curve was generated from measurements of serial dilutions of pooled cDNAs from individual POMC neurons. Cycle number was plotted against the normalized fluorescence intensity to visualize the PCR amplification and determine the amplification efficiencies. The amplification efficiency of a qPCR reaction for p110α, p110β and AMPK α2 was 91%, 91% and 99%, respectively. PCR products were analysed by melting curve analysis and agarose gel electrophoresis. All primer pairs were required to pass these quality-control checks. We used the comparative C t method (ΔΔ C t method) for quantification. Statistics Statistical analyses were performed using a paired or unpaired t -test as noted (Origin 8.5). The mean values were reported from the entire population tested (GraphPAD4.03 and Origin 8.5). Data were considered significantly different when the P value was <0.05. All statistical results are given as mean±s.e.m. How to cite this article: Lee, D. K. et al . Interplay between glucose and leptin signalling determines the strength of GABAergic synapses at POMC neurons. Nat. Commun. 6:6618 doi: 10.1038/ncomms7618 (2015).